ATR/Chk1/Smurf1 pathway determines cell fate after DNA damage by controlling RhoB abundance ATM- and RAD3-related (ATR)/Chk1 and ataxia–telangiectasia mutated (ATM)/Chk2 signalling pathways play critical roles in the DNA damage response. Here we report that the E3 ubiquitin ligase Smurf1 determines cell apoptosis rates downstream of DNA damage-induced ATR/Chk1 signalling by promoting degradation of RhoB, a small GTPase recognized as tumour suppressor by promoting death of transformed cells. We show that Smurf1 targets RhoB for degradation to control its abundance in the basal state. DNA damage caused by ultraviolet light or the alkylating agent methyl methanesulphonate strongly activates Chk1, leading to phosphorylation of Smurf1 that enhances its self-degradation, hence resulting in a RhoB accumulation to promote apoptosis. Suppressing RhoB levels by overexpressing Smurf1 or blocking Chk1-dependent Smurf1 self-degradation significantly inhibits apoptosis. Hence, our study unravels a novel ATR/Chk1/Smurf1/RhoB pathway that determines cell fate after DNA damage, and raises the possibility that aberrant upregulation of Smurf1 promotes tumorigenesis by excessively targeting RhoB for degradation. The ataxia–telangiectasia mutated (ATM) and ATM- and RAD3-related (ATR) kinases are master regulators orchestrating two distinct pathways, ATR/Chk1 and ATM/Chk2 signalling cascades in the DNA damage response. ATR/Chk1 signalling is usually activated by single-stranded DNA or bulky DNA lesions, whereas ATM/Chk2 pathway is activated by DNA double-strand breaks [1] , [2] . Despite the overlap between ATM- and ATR-regulated signalling pathways, ATM knockout mice are viable [3] , whereas ATR knockout leads to early embryonic lethality at E7.5 due to chromosomal fragmentation-induced apoptosis, presenting a critical role of ATR in maintaining genome integrity [4] . Consistently, knockout of Chk1 leads to the accumulation of DNA damage and apoptosis in ES cells, resulting in embryonic lethality at E6.5 (ref. 5 ), but Chk2-null mice appear normal [6] . In addition to maintaining the genome integrity during DNA replication, cell cycle transition and DNA repair, ATR/Chk1 signalling is also implicated in regulating apoptosis. Moreover, ATR/Chk1 may mediate apoptosis from different downstream pathways. For instance, Chk1 phosphorylates p73α, a p53-related transcription factor, to induce apoptosis in response to severe DNA damage [7] . Chk1 can also phosphorylate Lats2, which results in p21 degradation and leads to apoptosis [8] . Nevertheless, the underlying mechanism for ATR/Chk1 signalling in regulating apoptosis remains to be fully elucidated. Smurf1 (Smad ubiquitination regulatory factor 1) belongs to the HECT (homologous to the E6-AP carboxyl terminus) family of E3 ubiquitin ligases. It was first identified as a negative regulator of BMP (bone morphogenetic protein) signalling pathway by selectively downregulating the BMP pathway-specific Smad1 and Smad5 (ref. 9 ). Subsequent studies reveal that Smurf1 is also involved in regulating many other cellular activities, including bone morphology, cell polarity and motility, cell adhesion and TGFβ (transforming growth factor β)-induced epithelial-to-mesenchymal transition by targeting diverse substrates such as RUNXs, MEKK2, Prickle1, TRAF4, Talin head and small GTPase RhoA for ubiquitination [10] , [11] , [12] , [13] , [14] , [15] , [16] , [17] . Notably, Smurf1 is found upregulated in colon cancer and pancreatic cancer [18] , [19] , [20] , [21] , and its activity in mediating RhoA degradation is essential for cancer cell invasive activity [22] , [23] , [24] , [25] , demonstrating a pivotal role of Smurf1 in tumour progression. As a major group of the Ras superfamily GTP-binding proteins, the Rho family of small GTPases is recognized as key regulators of actin cytoskeleton dynamics [26] , [27] . Moreover, the Rho family small GTPases also regulate diverse cellular functions including cell cycle, gene expression, vesicle trafficking and cell polarity [28] , [29] . RhoA, RhoB and RhoC are 3 closely related Rho GTPases that share 85% amino-acid sequence identity. However, although RhoA, RhoB and RhoC all participate in inducing stress fibre formation, they may exert very distinct roles in different biological contexts [30] . In contrast to RhoA and RhoC that are frequently overexpressed in various human tumours, RhoB levels decrease in various types of cancer including lung cancer, gastric cancer, ovary carcinoma and head and neck cancer [31] , [32] , [33] , [34] , [35] , suggesting that RhoB suppresses tumorigenesis. Consistently, overexpression of RhoB potently inhibits tumour growth in nude mice [36] , [37] , [38] , whereas RhoB knockout in mice leads to increased susceptibility to chemical-induced skin carcinogenesis [39] . Mechanistic studies show that lack of RhoB significantly attenuates DNA damage-induced apoptosis of transformed cells [40] , and RhoB overexpression induces apoptosis in diverse cancer cell lines [41] , [42] , [43] , [44] , [45] , [46] , indicating that RhoB may exerts its tumour suppressor role through promoting cell apoptosis. In this study, we identify Smurf1 as a downstream effector in the ATR/Chk1 signalling pathway to determine the susceptibility of DNA damage-caused apoptosis by regulating RhoB levels. Activation of Chk1 after DNA damage mediates phosphorylation of Smurf1 to promote its self-degradation, resulting in an accumulation of RhoB to promote apoptosis. Excessive degradation of RhoB caused by upregulation of Smurf1 protects cancer cells from DNA damage-induced apoptosis, suggesting that Smurf1 is not only required for tumour metastasis by targeting RhoA for degradation as previously reported [12] , [16] , [25] , but may also be involved in tumour initiation by targeting RhoB for degradation. RhoB is a substrate for E3 ubiquitin ligase Smurf1 Our previous study showed that E3 ubiquitin ligase Smurf1 plays a key role in regulating cell polarity and protrusive activity through targeting small GTPase RhoA for degradation [13] . We then systematically investigated whether Smurf1 regulates other members of Rho family proteins. Interestingly, although RhoB and RhoC both share about 85% amino-acid sequence identity with RhoA [30] , wild-type Smurf1, but not catalytically inactive mutant Smurf1-C699A or its closest family member Smurf2, selectively decreased steady-state levels of RhoB but not RhoC ( Fig. 1a ). Meanwhile, overexpression of Smurf1 markedly downregulated endogenous RhoB levels ( Fig. 1b and Supplementary Fig. 1a ), whereas knockdown of Smurf1 significantly increased RhoB levels in both HeLa and HCT116 cells ( Fig. 1c and Supplementary Fig. 1b ). 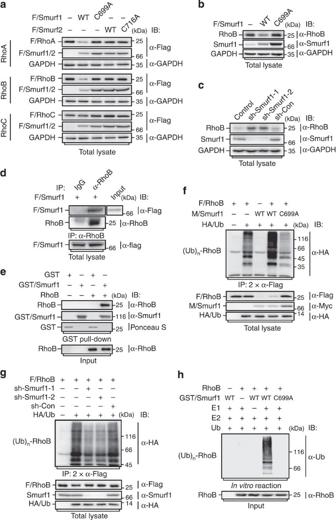Figure 1: Smurf1 targets RhoB for ubiquitination and degradation. (a) Overexpression of Smurf1 decreases protein levels of RhoA, RhoB, but not RhoC. HEK293T cells were transiently transfected with the indicated combinations of Flag-tagged RhoA (F/RhoA), RhoB (F/RhoB) or RhoC (F/RhoC) and Flag-tagged Smurf1 (F/Smurf1) or Smurf2 (F/Smurf2), wild-type (WT) or catalytically inactive mutants Smurf1-C699A (C699A) or Smurf2-C716A (C716A), respectively. Total cell lysates were subjected to immunoblotting (IB) to determine the protein levels. Levels of GAPDH were used as a loading control. (b) Smurf1 overexpression decreases endogenous RhoB protein levels. HeLa cells transduced with control lentivirus or lentivirus encoding F/Smurf1 (WT or C699A) were subjected to immunoblotting. (c) Knockdown of Smurf1 increases endogenous RhoB protein levels. HeLa cells transduced with lentivirus encoding control shRNA (sh-Con) or Smurf1 shRNA (sh-Smurf1-1 and sh-Smurf1-2) as indicated were subjected to immunoblotting. (d) Smurf1 interacts with endogenous RhoB proteins. Cell lysates from HeLa cells transduced with Flag-tagged Smurf1-C699A were subjected to anti-RhoB immunoprecipitation (IP) followed by immunoblotting with mouse anti-Flag to detect associated Smurf1-C699A. (e)In vitrointeraction between Smurf1 and RhoB. Bacterially expressed and purified RhoB protein and GST-tagged Smurf1 (GST/Smurf1) were subjected to GST pull-down assay as indicated. Associated RhoB and GST/Smurf1 were detected by immunoblotting with appropriate antibodies. GST was detected by Ponceau S staining. (f) Smurf1 promotes ubiquitination of RhoB. HEK293T cells transfected with indicated combinations of F/RhoB, Myc-tagged Smurf1 (Myc/Smurf1) (WT or C699A) and HA-tagged ubiquitin (HA/Ub) were treated with 10 μM MG-132 overnight before subjected to anti-Flag IP, eluted by boiling in 1% SDS, and then reprecipitated with anti-Flag antibody (2 × IP). Ubiquitin-conjugated RhoB [(Ub)n-RhoB] was detected by immunoblotting with anti-HA antibody. Expression of Myc/Smurf1, F/RhoB and HA/Ub were confirmed by immunoblotting the total cell lysates. (g) Knockdown of Smurf1 attenuates basal RhoB ubiquitination. HEK293T cells transfected with indicated combinations of F/RhoB, HA/Ub and small hairpin RNAs against Smurf1 were subjected to ubiquitination assay as described inf. (h) Smurf1 mediates ubiquitination of RhoB directlyin vitro. RhoB and GST/Smurf1 (WT or C699A) purified from bacteria were subjected to anin vitroubiquitination assay. Ubiquitinated RhoB was detected with anti-Ub antibody. Figure 1: Smurf1 targets RhoB for ubiquitination and degradation. ( a ) Overexpression of Smurf1 decreases protein levels of RhoA, RhoB, but not RhoC. HEK293T cells were transiently transfected with the indicated combinations of Flag-tagged RhoA (F/RhoA), RhoB (F/RhoB) or RhoC (F/RhoC) and Flag-tagged Smurf1 (F/Smurf1) or Smurf2 (F/Smurf2), wild-type (WT) or catalytically inactive mutants Smurf1-C699A (C699A) or Smurf2-C716A (C716A), respectively. Total cell lysates were subjected to immunoblotting (IB) to determine the protein levels. Levels of GAPDH were used as a loading control. ( b ) Smurf1 overexpression decreases endogenous RhoB protein levels. HeLa cells transduced with control lentivirus or lentivirus encoding F/Smurf1 (WT or C699A) were subjected to immunoblotting. ( c ) Knockdown of Smurf1 increases endogenous RhoB protein levels. HeLa cells transduced with lentivirus encoding control shRNA (sh-Con) or Smurf1 shRNA (sh-Smurf1-1 and sh-Smurf1-2) as indicated were subjected to immunoblotting. ( d ) Smurf1 interacts with endogenous RhoB proteins. Cell lysates from HeLa cells transduced with Flag-tagged Smurf1-C699A were subjected to anti-RhoB immunoprecipitation (IP) followed by immunoblotting with mouse anti-Flag to detect associated Smurf1-C699A. ( e ) In vitro interaction between Smurf1 and RhoB. Bacterially expressed and purified RhoB protein and GST-tagged Smurf1 (GST/Smurf1) were subjected to GST pull-down assay as indicated. Associated RhoB and GST/Smurf1 were detected by immunoblotting with appropriate antibodies. GST was detected by Ponceau S staining. ( f ) Smurf1 promotes ubiquitination of RhoB. HEK293T cells transfected with indicated combinations of F/RhoB, Myc-tagged Smurf1 (Myc/Smurf1) (WT or C699A) and HA-tagged ubiquitin (HA/Ub) were treated with 10 μM MG-132 overnight before subjected to anti-Flag IP, eluted by boiling in 1% SDS, and then reprecipitated with anti-Flag antibody (2 × IP). Ubiquitin-conjugated RhoB [(Ub)n-RhoB] was detected by immunoblotting with anti-HA antibody. Expression of Myc/Smurf1, F/RhoB and HA/Ub were confirmed by immunoblotting the total cell lysates. ( g ) Knockdown of Smurf1 attenuates basal RhoB ubiquitination. HEK293T cells transfected with indicated combinations of F/RhoB, HA/Ub and small hairpin RNAs against Smurf1 were subjected to ubiquitination assay as described in f . ( h ) Smurf1 mediates ubiquitination of RhoB directly in vitro . RhoB and GST/Smurf1 (WT or C699A) purified from bacteria were subjected to an in vitro ubiquitination assay. Ubiquitinated RhoB was detected with anti-Ub antibody. Full size image To test whether RhoB is a substrate of Smurf1, we first examined the interaction between Smurf1 and RhoB using Smurf1-C699A, the catalytically inactive form of Smurf1, to trap RhoB. Both endogenous and exogenous RhoB were found to associate with Smurf1-C699A ( Fig. 1d and Supplementary Fig. 1c ). In addition, in vitro glutathione S -transferase (GST) pull-down assay using bacterially expressed proteins showed that Smurf1 could directly bind RhoB ( Fig. 1e ). Next, we investigated the effect of Smurf1 on RhoB ubiquitination. Overexpression of wild-type Smurf1 but not Smurf1-C699A dramatically increased RhoB ubiquitination in vivo ( Fig. 1f ). Consistently, knockdown of Smurf1 significantly decreased the basal ubiquitination of RhoB ( Fig. 1g ), suggesting that endogenous Smurf1 targets RhoB for ubiquitination. We also performed in vitro ubiquitination assay using bacterially expressed RhoB and GST/Smurf1, and found that Smurf1 could directly catalyse ubiquitin conjugation of RhoB ( Fig. 1h ), confirming that RhoB is a direct substrate of Smurf1. Accordingly, co-expression of Smurf1 significantly decreased the half-life of RhoB, whereas knockdown of Smurf1 prolonged its half-life ( Supplementary Fig. 1d ). C2 domain is critical for Smurf1-mediated RhoB degradation Smurf1 consists of a C2 domain, two WW domains and a HECT domain, in which C2 domain is known as a phospholipid-binding domain, WW domains are used to interact with substrates containing PY motifs such as Smad1, and HECT is the E3 ligase catalytic domain. Our previous study showed that the C2 domain is critical for Smurf1 to bind RhoA [47] . Therefore, we examined the role of C2 domain in the interaction between Smurf1 and RhoB. Similar to RhoA, the C2 domain played an important role in interacting with RhoB as well ( Fig. 2a–c ). As shown in Fig. 2b , RhoB could associate with either full-length Smurf1 or Smurf1-truncated mutants that contain C2 and/or HECT domain, but not with Smurf1 mutant that only contains WW domains, in co-immunoprecipitation (IP) assay. In addition, GST pull-down assay using bacterially expressed proteins showed a strong interaction between RhoB and the C2 domain, indicating that the C2 domain of Smurf1 could directly bind RhoB ( Fig. 2c ). Intriguingly, deletion of the C2 domain completely blocked Smurf1-dependent exogenous and endogenous RhoB degradation ( Fig. 2d and Supplementary Fig. 2a ), it however retained partial activity towards mediating RhoB ubiquitination ( Fig. 2e ). Previous studies showed that in addition to regulating typical K48-linked ubiquitination, Smurf1 could also mediate unconventional ubiquitination through non-K48-linkage [48] , [49] . We therefore examined the chain linkage of ubiquitination of RhoB by using ubiquitin mutants R48 (only Lys48 mutated to Arg) and K48 (all Lys residues except Lys48 mutated to Arg). Interestingly, wild-type Smurf1-mediated RhoB ubiquitination using ubiquitin K48 mutant, whereas ΔC2 mutant and the HECT domain alone mediated RhoB ubiquitination using ubiquitin R48 mutant ( Supplementary Fig. 2b,c ), suggesting that deletion of C2 domain may change the pattern of Smurf1-mediated RhoB ubiquitination, likely owing to a conformational change of RhoB–Smurf1 complex upon the deletion of C2 domain. Hence, our results reveal a pivotal role of C2 domain in Smurf1-dependent RhoB degradation. 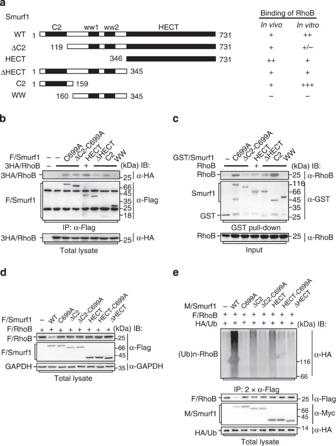Figure 2: The C2 domain of Smurf1 directly interacts with RhoB and is required for Smurf1-mediated RhoB ubiquitination and degradation. (a) Schematics of Smurf1 domains and truncated mutants. (b) Domain mapping for Smurf1 and RhoB interaction by co-immunoprecipitation assay. Cell lysates form HEK293T cells transfected with indicated combinations of triple HA-tagged RhoB (3HA/RhoB) and Flag-tagged Smurf1 (F/Smurf1) or its truncated mutants were subjected to anti-Flag IP followed by immunoblotting (IB) with rat anti-HA antibody to detect associated RhoB. (c)In vitrodomain mapping for Smurf1 and RhoB by GST pull-down assay. Bacterially expressed RhoB and GST-tagged Smurf1 (GST/Smurf1) or its truncated mutants were subjected to GST pull-down assay. Associated RhoB was detected by western blot with anti-RhoB antibody. (d) The C2 domain is required for Smurf1-mediated exogenous RhoB degradation. HEK293T cells transfected with combinations of Flag-tagged RhoB (F/RhoB) and F/Smurf1 (WT or indicated mutants) were subjected to immunoblotting. (e) Deletion of C2 domain attenuates Smurf1-mediated RhoB ubiquitination. HEK293T cells transfected with combinations of F/RhoB, HA/Ub and Myc/Smurf1 (WT or indicated mutants) were subjected to ubiquitination assay. Ubiquitinated RhoB was detected with anti-HA antibody. Figure 2: The C2 domain of Smurf1 directly interacts with RhoB and is required for Smurf1-mediated RhoB ubiquitination and degradation. ( a ) Schematics of Smurf1 domains and truncated mutants. ( b ) Domain mapping for Smurf1 and RhoB interaction by co-immunoprecipitation assay. Cell lysates form HEK293T cells transfected with indicated combinations of triple HA-tagged RhoB (3HA/RhoB) and Flag-tagged Smurf1 (F/Smurf1) or its truncated mutants were subjected to anti-Flag IP followed by immunoblotting (IB) with rat anti-HA antibody to detect associated RhoB. ( c ) In vitro domain mapping for Smurf1 and RhoB by GST pull-down assay. Bacterially expressed RhoB and GST-tagged Smurf1 (GST/Smurf1) or its truncated mutants were subjected to GST pull-down assay. Associated RhoB was detected by western blot with anti-RhoB antibody. ( d ) The C2 domain is required for Smurf1-mediated exogenous RhoB degradation. HEK293T cells transfected with combinations of Flag-tagged RhoB (F/RhoB) and F/Smurf1 (WT or indicated mutants) were subjected to immunoblotting. ( e ) Deletion of C2 domain attenuates Smurf1-mediated RhoB ubiquitination. HEK293T cells transfected with combinations of F/RhoB, HA/Ub and Myc/Smurf1 (WT or indicated mutants) were subjected to ubiquitination assay. Ubiquitinated RhoB was detected with anti-HA antibody. Full size image Lys6 and Lys7 residues are the ubiquitination sites We next identified the ubiquitin-conjugating site of RhoB in Smurf1-mediated ubiquitination. Since RhoA and RhoB are almost identical at their amino-terminal regions ( Fig. 3a ), and previous study showed that Smurf1 targets RhoA for ubiquitination on its Lys6 and Lys7 residues [12] , we hypothesized that Smurf1 may also catalyse the ubiquitin conjugation of RhoB on its Lys6 and Lys7. Indeed, similar to RhoA-K6,7R mutant [12] , RhoB-K6,7R was also resistant to Smurf1-induced degradation ( Fig. 3b ). Consistently, the Smurf1-dependent ubiquitination of RhoB was significantly attenuated by K6,7R mutation ( Fig. 3c ). Thus, our data demonstrate that Smurf1 indeed targets RhoB for ubiquitination at Lys6 and Lys7. 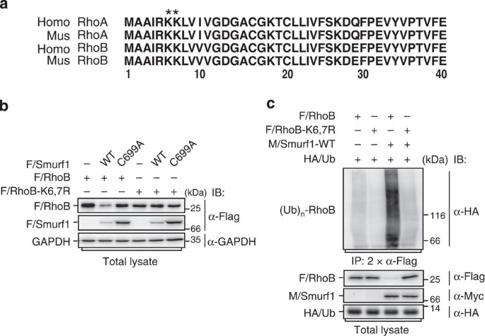Figure 3: Smurf1 mediates RhoB ubiquitination at its Lysines 6 and 7. (a) Amino-acid sequence alignment of RhoA and RhoB. Lys6 and Lys7 are indicated with asterisks. (b) Lysines 6 and 7 of RhoB are necessary for Smurf1-mediated RhoB degradation. HEK293T cells were transiently transfected with F/Smurf1 (WT or C699A) and Flag-tagged RhoB (F/RhoB) or RhoB-K6,7R mutant (F/RhoB-K6,7R). Steady-state protein levels were determined by immunoblotting. (c) Smurf1 targets RhoB ubiquitination at Lys6 and Lys7. HEK293T cells transfected with indicated combinations of HA/Ub, Myc/Smurf1 and Flag/RhoB or F/RhoB-K6,7R were subjected to ubiquitination assay. Ubiquitin-conjugated RhoB [(Ub)n-RhoB] was detected by immunoblotting with anti-HA antibody. Figure 3: Smurf1 mediates RhoB ubiquitination at its Lysines 6 and 7. ( a ) Amino-acid sequence alignment of RhoA and RhoB. Lys6 and Lys7 are indicated with asterisks. ( b ) Lysines 6 and 7 of RhoB are necessary for Smurf1-mediated RhoB degradation. HEK293T cells were transiently transfected with F/Smurf1 (WT or C699A) and Flag-tagged RhoB (F/RhoB) or RhoB-K6,7R mutant (F/RhoB-K6,7R). Steady-state protein levels were determined by immunoblotting. ( c ) Smurf1 targets RhoB ubiquitination at Lys6 and Lys7. HEK293T cells transfected with indicated combinations of HA/Ub, Myc/Smurf1 and Flag/RhoB or F/RhoB-K6,7R were subjected to ubiquitination assay. Ubiquitin-conjugated RhoB [(Ub)n-RhoB] was detected by immunoblotting with anti-HA antibody. Full size image RhoB degradation is not necessary for protrusive activity Since Smurf1-regulated RhoA degradation is important for cell protrusive activity [13] , we investigated whether Smurf1-mediated RhoB degradation has the similar function. Same as previously reported [13] , overexpression of wild-type Smurf1 but not Smurf1-C699A resulted in a large number of long protrusions in Mv1Lu epithelial cells ( Fig. 4a ). Interestingly, co-expression of RhoA-K6,7R strongly blocked Smurf1 overexpression-induced long protrusion formation, whereas co-expression of RhoB-K6,7R showed a much weaker blocking effect ( Fig. 4a,b ). Moreover, previous study showed that knockdown of Smurf1 causes HEK293T cells to lose their protrusions [13] . Simultaneously knockdown of RhoA but not RhoB rescued the cellular protrusions in Smurf1 knocked-down cells ( Fig. 4c ). In addition, overexpression of either RhoA-K6,7R or RhoB-K6,7R did not affect Smurf1-mediated degradation of RhoA or RhoB, indicating that the K6,7R mutant of RhoA or RhoB is not functioning as a dominant-negative form of substrate ( Supplementary Fig. 3a–d ). These results suggest that Smurf1 regulates protrusive activity through mediating RhoA but not RhoB degradation. 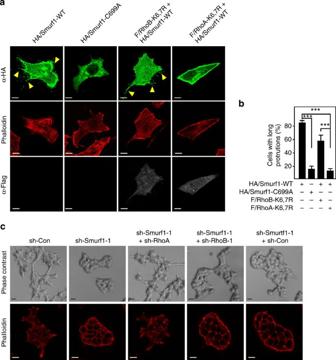Figure 4: Smurf1-mediated RhoB degradation is dispensable for regulation of cell protrusive activity. (a,b) RhoA-K6,7R but not RhoB-K6,7R blocks Smurf1-induced long protrusion formation. Mv1Lu cells were transfected with HA-tagged Smurf1 (HA/Smurf1), wild-type (WT) or catalytically inactive mutant (C699A), with or without Flag-tagged RhoA-K6,7R (F/RhoA-K6,7R) or RhoB-K6,7R (F/RhoB-K6,7R) as indicated. The cells were subjected to immunofluorescence assay with appropriate antibodies to examine the protein expression 24 h after transfection and Texas red conjugated Phalloidin was used to visualize F-actin (a). The scale bars indicate 5 μm. The percentage of Mv1Lu cells with long protrusions were quantified and plotted inb. A minimum of 100 cells were scored for each experiment and data are represented as mean±s.d. of three independent experiments. Data are assessed by one-way analysis of variance and Tukey’s HSD post test after arcsine transformation. ***P<0.001. (c) Knockdown of RhoA but not RhoB rescues the morphological change and actin cytoskeleton rearrangements caused by reducing Smurf1 levels. HEK293T cells were transfected with indicated combinations of small hairpin RNAs against Smurf1 (sh-Smurf1-1), RhoA (sh-RhoA) or RhoB (sh-RhoB-1) as indicated. The cells were visualized 48 h later by phase contrast microscopy (top) or Texas red-phalloidin staining (bottom). The scale bars indicate 20 μm. Figure 4: Smurf1-mediated RhoB degradation is dispensable for regulation of cell protrusive activity. ( a , b ) RhoA-K6,7R but not RhoB-K6,7R blocks Smurf1-induced long protrusion formation. Mv1Lu cells were transfected with HA-tagged Smurf1 (HA/Smurf1), wild-type (WT) or catalytically inactive mutant (C699A), with or without Flag-tagged RhoA-K6,7R (F/RhoA-K6,7R) or RhoB-K6,7R (F/RhoB-K6,7R) as indicated. The cells were subjected to immunofluorescence assay with appropriate antibodies to examine the protein expression 24 h after transfection and Texas red conjugated Phalloidin was used to visualize F-actin ( a ). The scale bars indicate 5 μm. The percentage of Mv1Lu cells with long protrusions were quantified and plotted in b . A minimum of 100 cells were scored for each experiment and data are represented as mean±s.d. of three independent experiments. Data are assessed by one-way analysis of variance and Tukey’s HSD post test after arcsine transformation. *** P <0.001. ( c ) Knockdown of RhoA but not RhoB rescues the morphological change and actin cytoskeleton rearrangements caused by reducing Smurf1 levels. HEK293T cells were transfected with indicated combinations of small hairpin RNAs against Smurf1 (sh-Smurf1-1), RhoA (sh-RhoA) or RhoB (sh-RhoB-1) as indicated. The cells were visualized 48 h later by phase contrast microscopy (top) or Texas red-phalloidin staining (bottom). The scale bars indicate 20 μm. Full size image Smurf1-mediated RhoB degradation inhibits apoptosis It has been reported that RhoB plays an important role in DNA damage-induced apoptosis, and functions as a tumour suppressor [46] . In agreement with previous reports, knockdown of RhoB significantly decreased ultraviolet or methyl methanesulphonate (MMS)-induced apoptosis in HeLa cells ( Fig. 5a and Supplementary Fig. 4a,b ). In addition, overexpression of either wild-type RhoB or RhoB-K6,7R enhanced the apoptotic effects in a dose-dependent manner ( Fig. 5b and Supplementary Fig. 4c,d ). The protein levels of endogenous and exogenous RhoB were validated by western blot ( Supplementary Fig. 4e,f ). We therefore asked whether Smurf1-dependent RhoB degradation is involved in regulating apoptosis in response to DNA damage. To test this possibility, we first examined the levels of Smurf1 and RhoB in HeLa cells in response to ultraviolet or MMS treatment. Remarkably, Smurf1 protein levels significantly decreased after lethal dose (80 J m −2 ) ultraviolet or MMS treatment, with a corresponding increase of RhoB ( Fig. 5c,d ), whereas low-dose (10 J m −2 ) ultraviolet radiation, which did not induce significant levels of apoptosis in HeLa cells, did not change the protein levels of Smurf1 and RhoB ( Fig. 5c ). The downregulation of Smurf1 and correlated increase of RhoB in response to ultraviolet or MMS treatment could also be observed in various other cell lines including human colon cancer HCT116, human hepatocellular carcinoma HepG2, human non-small lung cancer A549 and human breast cancer MCF-7 cells ( Supplementary Fig. 5a,b ), suggesting that changes of Smurf1 and RhoB protein levels may be correlated with apoptosis. However, treatment of cisplatin or doxorubicin (Dox), two other commonly used DNA-damaging agents, did not affect either Smurf1 or RhoB protein levels ( Supplementary Fig. 5c,d ). 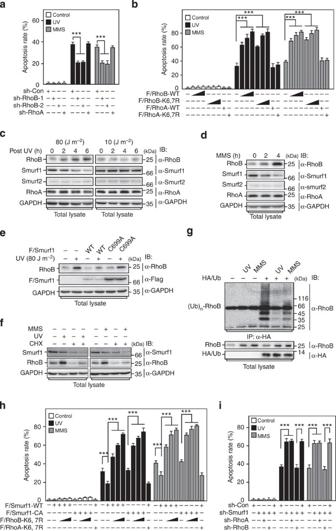Figure 5: Smurf1 inhibits ultraviolet or MMS-induced apoptosis through downregulating RhoB. (a) RhoB is required for ultraviolet or MMS-induced apoptosis. HeLa cells transduced with lentivirus encoding indicated small hairpin RNAs were subjected to flow cytometry assay 24 h after 80 J m−2ultraviolet or 0.5 mM MMS treatment. Data of three independent experiments were assessed by one-way analysis of variance and Tukey’s HSD post test after arcsine transformation and represented as mean±s.d. ***P<0.001. (b) RhoB dose dependently enhances ultraviolet or MMS-induced apoptosis. HeLa cells with overexpression of F/RhoB or F/RhoA (WT or K6,7R) were treated and analysed same as ina. Data assessment is same as ina. ***P<0.001. (c,d) Lethal dose of ultraviolet or MMS treatment upregulates RhoB levels and downregulates Smurf1 levels. HeLa cells were lysed at indicated time points after treatment of ultraviolet (80 or 10 J m−2) (c) or 0.5 mM MMS (d) before subjected to immunoblotting. (e) Overexpression of Smurf1 attenuates ultraviolet-induced RhoB upregulation. HeLa cells with overexpression of F/Smurf1 (WT or C699A) were subjected to immunoblotting 4 h after irradiated with 80 J m−2ultraviolet. (f) Ultraviolet or MMS treatment stabilizes RhoB. HeLa cells pretreated with or without cycloheximide (CHX, 3.5 μM) 0.5 h before treated with ultraviolet (80 J m−2) or MMS (0.5 mM) were lysed 4 h later and subjected to immunoblotting. (g) Ultraviolet or MMS treatment attenuates endogenous RhoB ubiquitination. HeLa cells transduced with lentivirus encoding HA/Ub were lysed 6 h after ultraviolet or MMS treatment before subjected to immunoprecipitation with anti-HA antibody. Ubiquitinated RhoB was detected with anti-RhoB antibody. (h) Smurf1 suppresses ultraviolet or MMS-induced apoptosis via downregulating RhoB. HeLa cells with overexpression of indicated combination of F/Smurf1 (WT or C699A), F/RhoA-K6,7R or F/RhoB-K6,7R were treated and analysed same as ina. Data assessment is same as ina. ***P<0.001. (i) Simultaneously knocking down RhoB suppresses Smurf1 knockdown-enhanced apoptosis. HeLa cells transduced with lentivirus encoding indicated small hairpin RNAs were treated same as inabefore subjected to flow cytometry assay. Data were assessed same as ina. ***P<0.001. Figure 5: Smurf1 inhibits ultraviolet or MMS-induced apoptosis through downregulating RhoB. ( a ) RhoB is required for ultraviolet or MMS-induced apoptosis. HeLa cells transduced with lentivirus encoding indicated small hairpin RNAs were subjected to flow cytometry assay 24 h after 80 J m −2 ultraviolet or 0.5 mM MMS treatment. Data of three independent experiments were assessed by one-way analysis of variance and Tukey’s HSD post test after arcsine transformation and represented as mean±s.d. *** P <0.001. ( b ) RhoB dose dependently enhances ultraviolet or MMS-induced apoptosis. HeLa cells with overexpression of F/RhoB or F/RhoA (WT or K6,7R) were treated and analysed same as in a . Data assessment is same as in a . *** P <0.001. ( c , d ) Lethal dose of ultraviolet or MMS treatment upregulates RhoB levels and downregulates Smurf1 levels. HeLa cells were lysed at indicated time points after treatment of ultraviolet (80 or 10 J m −2 ) ( c ) or 0.5 mM MMS ( d ) before subjected to immunoblotting. ( e ) Overexpression of Smurf1 attenuates ultraviolet-induced RhoB upregulation. HeLa cells with overexpression of F/Smurf1 (WT or C699A) were subjected to immunoblotting 4 h after irradiated with 80 J m −2 ultraviolet. ( f ) Ultraviolet or MMS treatment stabilizes RhoB. HeLa cells pretreated with or without cycloheximide (CHX, 3.5 μM) 0.5 h before treated with ultraviolet (80 J m −2 ) or MMS (0.5 mM) were lysed 4 h later and subjected to immunoblotting. ( g ) Ultraviolet or MMS treatment attenuates endogenous RhoB ubiquitination. HeLa cells transduced with lentivirus encoding HA/Ub were lysed 6 h after ultraviolet or MMS treatment before subjected to immunoprecipitation with anti-HA antibody. Ubiquitinated RhoB was detected with anti-RhoB antibody. ( h ) Smurf1 suppresses ultraviolet or MMS-induced apoptosis via downregulating RhoB. HeLa cells with overexpression of indicated combination of F/Smurf1 (WT or C699A), F/RhoA-K6,7R or F/RhoB-K6,7R were treated and analysed same as in a . Data assessment is same as in a . *** P <0.001. ( i ) Simultaneously knocking down RhoB suppresses Smurf1 knockdown-enhanced apoptosis. HeLa cells transduced with lentivirus encoding indicated small hairpin RNAs were treated same as in a before subjected to flow cytometry assay. Data were assessed same as in a . *** P <0.001. Full size image Interestingly, the ultraviolet or MMS treatment-caused decrease of Smurf1 was not due to downregulation of its messenger RNA (mRNA) levels ( Supplementary Fig. 6a ). In agreement with previous reports that transcription of RhoB can be quickly induced by DNA-damaging stresses [50] , [51] , we observed that RhoB mRNA levels increased to 1.5-fold after ultraviolet or MMS treatment ( Supplementary Fig. 6b ). Nevertheless, it is unlikely enough to cause such a dramatic increase of RhoB protein levels. Hence, we tested whether attenuation of the Smurf1-mediated RhoB degradation is required for the upregulation of RhoB induced by ultraviolet or MMS. Indeed, exogenous expression of Smurf1 significantly inhibited the increase of RhoB in ultraviolet or MMS-treated cells ( Fig. 5e and Supplementary Fig. 6c ). We further validated the contribution of stabilization of RhoB in its upregulation by blocking protein translation or gene transcription using cycloheximide or actinomycin, respectively. Indeed, the protein levels of RhoB in cells treated with ultraviolet or MMS were significantly higher than that in cells without ultraviolet or MMS treatment even when protein translation or gene transcription had been blocked ( Fig. 5f and Supplementary Fig. 6d–f ). Moreover, treatment of ultraviolet or MMS significantly attenuated basal ubiquitination of RhoB and increased its half-life ( Fig. 5g , Supplementary Fig. 6g,h ), confirming that increasing the protein stability of RhoB plays a key role in upregulation of RhoB in response to ultraviolet or MMS treatment. Next, we examined the roles of Smurf1 in regulating ultraviolet or MMS-triggered apoptosis. As expected, overexpression of wild-type Smurf1 but not Smurf1-C699A significantly reduced apoptotic rates of HeLa cells after ultraviolet radiation or MMS treatment ( Fig. 5h and Supplementary Fig. 7a,b ). To determine whether reduced apoptosis caused by Smurf1 overexpression is through enhancing RhoB degradation, we co-expressed RhoB-K6,7R to do the rescue experiments. Indeed, co-expression of RhoB-K6,7R rescued the ultraviolet or MMS treatment-induced apoptosis in a dose-dependent manner, whereas co-expression of RhoA-K6,7R had no rescue effect ( Fig. 5h and Supplementary Fig. 7a,b ). Meanwhile, knockdown of Smurf1 markedly enhanced ultraviolet or MMS treatment-induced apoptosis, and simultaneously knocking down RhoB but not RhoA significantly decreased the apoptotic rates upregulated by Smurf1 knockdown ( Fig. 5i and Supplementary Fig. 7c,d ). The corresponding levels of RhoB were validated by immunoblotting (IB) ( Supplementary Fig. 8a-c ). These results demonstrate that Smurf1 regulates the apoptotic susceptibility to ultraviolet or MMS-induced DNA damage via controlling RhoB protein levels. ATR/Chk1 signalling promotes Smurf1 autodegradation We next investigated the mechanism by which Smurf1 is downregulated in response to DNA damage. Since the downregulation of Smurf1 caused by ultraviolet or MMS treatment was not due to the decrease of its mRNA levels ( Supplementary Fig. 6a ), we examined whether it is through protein degradation. Indeed, the proteasome inhibitor MG-132 could effectively protect Smurf1 from ultraviolet or MMS-induced downregulation ( Fig. 6a ), indicating that the decrease of Smurf1 after ultraviolet or MMS treatment is via proteasome-dependent degradation pathway. As previous report showed that Smurf1 could target itself for ubiquitination [52] , we further tested whether the decrease of Smurf1 is through self-degradation. Remarkably, wild-type Smurf1 but not Smurf1-C699A mutant was decreased after ultraviolet or MMS treatment ( Fig. 6b,c ), indicating that the ultraviolet or MMS treatment-induced downregulation of Smurf1 is dependent on its E3 ligase catalytic activity. Correspondingly, ultraviolet or MMS treatment drastically enhanced ubiquitination of wild-type Smurf1 but not catalytic inactive mutant Smurf1-C699A ( Fig. 6d ), confirming that downregulation of Smurf1 caused by ultraviolet or MMS is through enhancing its self-ubiquitination. 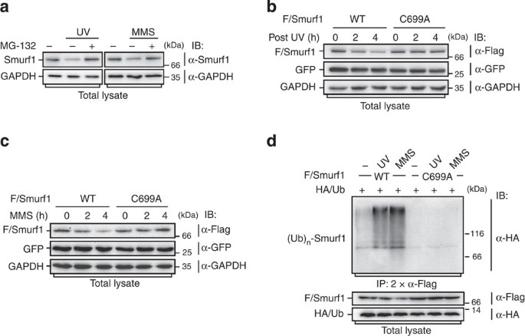Figure 6: Ultraviolet or MMS treatment promotes Smurf1 auto-ubiquitination and self-degradation. (a) Ultraviolet or MMS treatment downregulates Smurf1 through proteasome pathway. HeLa cells were pretreated with or without MG-132 (20 μM) 2 h before treated with ultraviolet (80 J m−2) or MMS (0.5 mM). The cells were then lysed 4 h after ultraviolet irradiation or MMS treatment and subjected to immunoblotting assay. (b) Ultraviolet irradiation-induced Smurf1 downregulation is dependent on its E3 ligase activity. HeLa cells transduced with lentivirus encoding Flag-tagged Smurf1 (WT or C699A) were treated with 80 J m−2ultraviolet lysed at indicated time points after ultraviolet irradiation, and then subjected to western blot assay. GFP and GAPDH levels were used as transfection and loading controls, respectively. (c) MMS treatment-induced Smurf1 downregulation is dependent on its E3 ligase activity. Same as inbexcept cells were treated with MMS (0.5 mM) instead of ultraviolet irradiation. (d) Ultraviolet irradiation or MMS treatment promotes Smurf1 auto-ubiquitination. HEK293T cells transfected with Flag-tagged Smurf1 (WT or C699A) together with HA-tagged ubiquitin (HA/Ub) as indicated were subjected to ubiquitination assay. Ubiquitin-conjugated Smurf1 [(Ub)n-Smurf1] was detected by immunoblotting with anti-HA antibody. Figure 6: Ultraviolet or MMS treatment promotes Smurf1 auto-ubiquitination and self-degradation. ( a ) Ultraviolet or MMS treatment downregulates Smurf1 through proteasome pathway. HeLa cells were pretreated with or without MG-132 (20 μM) 2 h before treated with ultraviolet (80 J m −2 ) or MMS (0.5 mM). The cells were then lysed 4 h after ultraviolet irradiation or MMS treatment and subjected to immunoblotting assay. ( b ) Ultraviolet irradiation-induced Smurf1 downregulation is dependent on its E3 ligase activity. HeLa cells transduced with lentivirus encoding Flag-tagged Smurf1 (WT or C699A) were treated with 80 J m −2 ultraviolet lysed at indicated time points after ultraviolet irradiation, and then subjected to western blot assay. GFP and GAPDH levels were used as transfection and loading controls, respectively. ( c ) MMS treatment-induced Smurf1 downregulation is dependent on its E3 ligase activity. Same as in b except cells were treated with MMS (0.5 mM) instead of ultraviolet irradiation. ( d ) Ultraviolet irradiation or MMS treatment promotes Smurf1 auto-ubiquitination. HEK293T cells transfected with Flag-tagged Smurf1 (WT or C699A) together with HA-tagged ubiquitin (HA/Ub) as indicated were subjected to ubiquitination assay. Ubiquitin-conjugated Smurf1 [(Ub)n-Smurf1] was detected by immunoblotting with anti-HA antibody. Full size image Since protein kinases ATM and ATR (ATM and Rad3 related) are master regulators of DNA damage response [1] , we detected whether ATM/ATR signalling is required for Smurf1 downregulation in response to DNA damage. Strikingly, ATM/ATR inhibitor caffeine significantly blocked the decrease of Smurf1 and the corresponding increase of RhoB caused by ultraviolet or MMS treatment ( Fig. 7a and Supplementary Fig. 9a ), suggesting that ATM/ATR signalling is involved in regulating the stability of Smurf1. Further examination using small hairpin RNAs to specifically knock down ATM or ATR indicated that ATR but not ATM is the upstream regulator for Smurf1 downregulation ( Fig. 7b and Supplementary Fig. 9b ). Since the checkpoint kinase 1 (Chk1) and checkpoint kinase 2 (Chk2) are key downstream kinases of ATM/ATR signalling in DNA damage response [1] , [2] , we next investigated whether Chk1 and/or Chk2 are required for promoting Smurf1 self-degradation. Significantly, treatment of Chk1 inhibitor but not Chk2 inhibitor effectively blocked ultraviolet or MMS-caused decrease of Smurf1 and increase of RhoB ( Fig. 7c and Supplementary Fig. 9c ). We further confirmed that it is Chk1 but not Chk2 responsible for downregulating Smurf1 in response to DNA damage by specifically knocking down Chk1 or Chk2 ( Fig. 7d,e and Supplementary Fig. 9d,e ). Furthermore, overexpression of Chk1-D130A, a dominant-negative form of Chk1, strongly inhibited the downregulation of Smurf1 and upregulation of RhoB caused by ultraviolet or MMS treatment ( Fig. 7f and Supplementary Fig. 9f ), which further confirmed that the activity of Chk1 is necessary to promote Smurf1 self-degradation. The efficiency of cells expressing Chk1-D130A was confirmed by immunofluorescence assay ( Supplementary Fig. 9g ). Moreover, the necessity of Chk1 activity in downregulating Smurf1 levels after ultraviolet or MMS treatment was also confirmed in HCT116 colorectal cancer cells ( Supplementary Fig. 10a-e and Supplementary Fig. 11a–e ). Interestingly, we examined the phosphorylation of Chk1 and Chk2 and found that treatment of ultraviolet or MMS strongly activated Chk1, whereas cisplatin or Dox treatment potently activated Chk2 but not Chk1 ( Supplementary Fig. 12a,b ). It is noteworthy that Smurf1 is upregulated in various types of cancer [18] , [19] , [20] , [21] , and Chk1 is frequently activated in cancer cells, however, the levels of activated chk1 in cancer cells are dramatically lower than that in cells after ultraviolet or MMS treatment ( Supplementary Fig. 12c,d ), suggesting that a higher kinase activity level of Chk1 are required for promoting Smurf1 self-degradation. 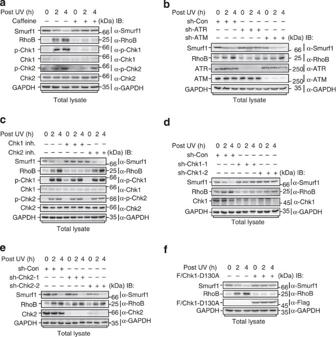Figure 7: Ultraviolet irradiation promotes Smurf1 self-degradation through activating ATR/Chk1 signalling pathway. (a) Inactivation of ATM/ATR prevents Smurf1 downregulation and RhoB upregulation after ultraviolet irradiation. HeLa cells were pretreated with or without caffeine (3 mM) for 1 h before irradiated with 80 J m−2ultraviolet. Endogenous levels of Smurf1 and RhoB at indicated time points after ultraviolet irradiation were examined by immunoblotting. (b) Knockdown of ATR dampened Smurf1 downregulation and RhoB upregulation after ultraviolet irradiation. HeLa cells transduced with lentivirus encoding control shRNA or small hairpin RNAs (shRNAs) against ATR or ATM were lysed at indicated time points after ultraviolet irradiation and subjected to immunoblotting. (c) Chk1 activity is required for ultraviolet-induced Smurf1 downregulation and RhoB upregulation. HeLa cells were pretreated with or without Chk1 inhibitor UCN-01 (Chk1 inh, 0.1 μM) or Chk2 inhibitor-II (Chk2 inh, 5 μM) for 1 h before irradiated with 80 J m−2ultraviolet. Cells were then lysed at indicated time points after ultraviolet treatment and subjected to immunoblotting assay. (d,e) Knockdown of Chk1 but not Chk2 inhibits ultraviolet-induced Smurf1 downregulation and RhoB upregulation. HeLa cells transduced with lentivirus encoding control shRNA or shRNAs against Chk1 (d) or Chk2 (e) were lysed at indicated time points after 80 J m−2ultraviolet irradiation, and then subjected to immunoblotting assay. (f) Overexpression of dominant-negative form of Chk1 blocks ultraviolet-induced Smurf1 downregulation and RhoB upregulation. HeLa cells transduced with control lentivirus or lentivirus encoding Flag-tagged kinase-dead mutant Chk1-D130A (F/Chk1-D130A) were irradiated with ultraviolet (80 J m−2), lysed at indicated time points after the irradiation, and then subjected to immunoblotting. Figure 7: Ultraviolet irradiation promotes Smurf1 self-degradation through activating ATR/Chk1 signalling pathway. ( a ) Inactivation of ATM/ATR prevents Smurf1 downregulation and RhoB upregulation after ultraviolet irradiation. HeLa cells were pretreated with or without caffeine (3 mM) for 1 h before irradiated with 80 J m −2 ultraviolet. Endogenous levels of Smurf1 and RhoB at indicated time points after ultraviolet irradiation were examined by immunoblotting. ( b ) Knockdown of ATR dampened Smurf1 downregulation and RhoB upregulation after ultraviolet irradiation. HeLa cells transduced with lentivirus encoding control shRNA or small hairpin RNAs (shRNAs) against ATR or ATM were lysed at indicated time points after ultraviolet irradiation and subjected to immunoblotting. ( c ) Chk1 activity is required for ultraviolet-induced Smurf1 downregulation and RhoB upregulation. HeLa cells were pretreated with or without Chk1 inhibitor UCN-01 (Chk1 inh, 0.1 μM) or Chk2 inhibitor-II (Chk2 inh, 5 μM) for 1 h before irradiated with 80 J m −2 ultraviolet. Cells were then lysed at indicated time points after ultraviolet treatment and subjected to immunoblotting assay. ( d , e ) Knockdown of Chk1 but not Chk2 inhibits ultraviolet-induced Smurf1 downregulation and RhoB upregulation. HeLa cells transduced with lentivirus encoding control shRNA or shRNAs against Chk1 ( d ) or Chk2 ( e ) were lysed at indicated time points after 80 J m −2 ultraviolet irradiation, and then subjected to immunoblotting assay. ( f ) Overexpression of dominant-negative form of Chk1 blocks ultraviolet-induced Smurf1 downregulation and RhoB upregulation. HeLa cells transduced with control lentivirus or lentivirus encoding Flag-tagged kinase-dead mutant Chk1-D130A (F/Chk1-D130A) were irradiated with ultraviolet (80 J m −2 ), lysed at indicated time points after the irradiation, and then subjected to immunoblotting. Full size image Chk1 phosphorylates Smurf1 in response to DNA damage To investigate whether Smurf1 is a substrate of Chk1, we first examined the interaction between Chk1 and Smurf1. Endogenous Smurf1 was able to co-immunoprecipitate with Chk1 ( Fig. 8a ), and the interaction between Smurf1 and Chk1 was significantly enhanced by ultraviolet or MMS treatment ( Fig. 8b ). Remarkably, neither binding of Smurf1 to Chk2 nor binding of Smurf2 to Chk1 could be detected, indicating that Smurf1 specifically interacted with Chk1 ( Fig. 8c ). We next examined the location where Chk1 binds Smurf1 by subcellular fractionation assay. Smurf1 is located in both nucleus and cytoplasm, whereas Chk1 is mainly in nucleus and RhoB is in cytosol ( Supplementary Fig. 13a ), and Smurf1 interacts with Chk1 in nucleus ( Supplementary Fig. 13b ). Ultraviolet or MMS treatment induces downregulation of Smurf1 in both nucleus and cytosol ( Supplementary Fig. 13a ), indicating that although Chk1-induced Smurf1 auto-ubiquitination might mainly occur in nucleus, it drains the pool of Smurf1. Furthermore, we performed GST pull-down assay using bacterially expressed proteins and found that Chk1 could directly interact with Smurf1 in vitro ( Fig. 8d ). 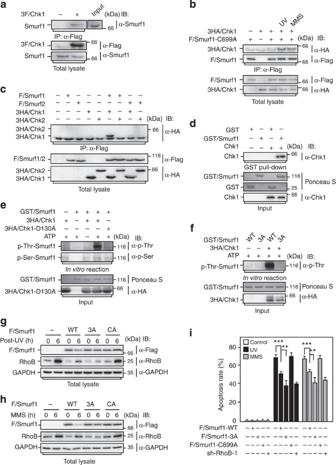Figure 8: Chk1 promotes Smurf1 self-degradation by phosphorylating Smurf1. (a) Chk1 interacts with endogenous Smurf1. HeLa cells transduced with control lentivirus or lentivirus encoding triple Flag-tagged Chk1 (3F/Chk1) were subjected to co-immunoprecipitation assay to detect associated Smurf1. (b) Ultraviolet or MMS treatment enhances the interaction between Smurf1 and Chk1. HeLa cells transduced with lentivirus encoding F/Smurf1-C699A and 3HA-tagged (3HA/Chk1) as indicated were treated with ultraviolet (80 J m−2) or MMS (0.5 mM), and subjected to co-IP assay 30 min later to detect associated Chk1. (c) Chk1 but not Chk2 specifically interacts with Smurf1. HEK293T cells transfected with indicated combinations of F/Smurf1-C699A, F/Smurf2-C716A, 3HA/Chk1, and 3HA/Chk2 were subjected to co-IP assay. (d)In vitrointeraction between Chk1 and Smurf1. Chk1 and GST/Smurf1 purified from bacteria were subjected to GST pull-down assay. Associated Chk1 was determined by immunoblotting with anti-Chk1 antibody. GST/Smurf1 and GST were detected by Ponceau S staining. (e) Chk1 phosphorylates Smurf1 at its threonine residues.In vitrokinase assay was carried out by incubating GST/Smurf1 with 3HA/Chk1 immunoprecipitated from MMS (0.5 mM, 2 h) treated HeLa cells. Phosphorylation of Smurf1 was detected by immunoblotting using phosphothreonine or phospho-serine antibodies. (f) Chk1 phosphorylates Smurf1 at Thr145, Thr161 and Thr682. GST/Smurf1, WT or T145,161,682A mutant (3A), were used to performin vitrokinase assay same as ine. (g,h) Phosphorylation of Smurf1 by Chk1 is necessary for ultraviolet or MMS-induced down-regulation of Smurf1. HeLa cells transduced with control lentivirus or lentivirus encoding F/Smurf1 (WT, 3A or C699A) were subjected to immunoblotting at indicated time points after treated with 80 J m−2ultraviolet (g) or 0.5 mM MMS (h). (i) Smurf1-3A has more potent effect on suppressing ultraviolet or MMS-induced apoptosis. HeLa cells transduced with control lentivirus or lentivirus encoding F/Smurf1 (WT, 3A or C699A) were treated with 80 J m−2ultraviolet or 0.5 mM MMS and then subjected to flow cytometry assay 32 h after the treatment. Data of three independent experiments were assessed by one-way analysis of variance and Tukey’s HSD post test after arcsine transformation and represented as mean±s.d. **P<0.01, ***P<0.001. Figure 8: Chk1 promotes Smurf1 self-degradation by phosphorylating Smurf1. ( a ) Chk1 interacts with endogenous Smurf1. HeLa cells transduced with control lentivirus or lentivirus encoding triple Flag-tagged Chk1 (3F/Chk1) were subjected to co-immunoprecipitation assay to detect associated Smurf1. ( b ) Ultraviolet or MMS treatment enhances the interaction between Smurf1 and Chk1. HeLa cells transduced with lentivirus encoding F/Smurf1-C699A and 3HA-tagged (3HA/Chk1) as indicated were treated with ultraviolet (80 J m −2 ) or MMS (0.5 mM), and subjected to co-IP assay 30 min later to detect associated Chk1. ( c ) Chk1 but not Chk2 specifically interacts with Smurf1. HEK293T cells transfected with indicated combinations of F/Smurf1-C699A, F/Smurf2-C716A, 3HA/Chk1, and 3HA/Chk2 were subjected to co-IP assay. ( d ) In vitro interaction between Chk1 and Smurf1. Chk1 and GST/Smurf1 purified from bacteria were subjected to GST pull-down assay. Associated Chk1 was determined by immunoblotting with anti-Chk1 antibody. GST/Smurf1 and GST were detected by Ponceau S staining. ( e ) Chk1 phosphorylates Smurf1 at its threonine residues. In vitro kinase assay was carried out by incubating GST/Smurf1 with 3HA/Chk1 immunoprecipitated from MMS (0.5 mM, 2 h) treated HeLa cells. Phosphorylation of Smurf1 was detected by immunoblotting using phosphothreonine or phospho-serine antibodies. ( f ) Chk1 phosphorylates Smurf1 at Thr145, Thr161 and Thr682. GST/Smurf1, WT or T145,161,682A mutant (3A), were used to perform in vitro kinase assay same as in e . ( g , h ) Phosphorylation of Smurf1 by Chk1 is necessary for ultraviolet or MMS-induced down-regulation of Smurf1. HeLa cells transduced with control lentivirus or lentivirus encoding F/Smurf1 (WT, 3A or C699A) were subjected to immunoblotting at indicated time points after treated with 80 J m −2 ultraviolet ( g ) or 0.5 mM MMS ( h ). ( i ) Smurf1-3A has more potent effect on suppressing ultraviolet or MMS-induced apoptosis. HeLa cells transduced with control lentivirus or lentivirus encoding F/Smurf1 (WT, 3A or C699A) were treated with 80 J m −2 ultraviolet or 0.5 mM MMS and then subjected to flow cytometry assay 32 h after the treatment. Data of three independent experiments were assessed by one-way analysis of variance and Tukey’s HSD post test after arcsine transformation and represented as mean±s.d. ** P <0.01, *** P <0.001. Full size image Next, we carried out in vitro phosphorylation assay to examine whether Chk1 can phosphorylate Smurf1. Strikingly, strong phosphorylation of threonine residue(s) in Smurf1 was observed by using a phospho-Thr specific antibody when GST/Smurf1 was incubated with wild-type Chk1 but not Chk1-D130A in the in vitro reaction, whereas no significant phosphorylation of serine residue in Smurf1 could be detected ( Fig. 8e ). Using matrix-assisted laser desorption/ionization time-of-flight mass spectrometry (MALDI-TOF-MS), we identified that Thr145, Thr161 and Thr682 of Smurf1 could be phosphorylated by Chk1 ( Supplementary Fig. 14 ). We next used Smurf1-3A, a mutant with Thr145, Thr161 and Thr682 mutated to alanines, to perform the in vitro phosphorylation assay. As expected, point mutations of these three threonine residues to alanine totally abolished the Chk1-mediated phosphorylation of Smurf1 ( Fig. 8f ), confirming that the phosphorylation sites for Chk1 in Smurf1 are at Thr145, Thr161 and Thr682. To verify these phosphorylation sites in cells, we immunoprecipitated Flag-tagged Smurf1-C699A from cells treated with or without ultraviolet or MMS and then subjected it to mass spectrometry assays. Indeed, we found that all the three sites, Thr145, Thr161 and Thr682, could be phosphorylated after ultraviolet or MMS treatment ( Supplementary Fig. 15a,b ), whereas no phosphorylation of these sites could be detected in cells without treatment. We next assessed the role of Chk1-mediated phosphorylation in ATR/Chk1 signalling-induced Smurf1 downregulation by examining the changes of Smurf1-3A protein levels in response to ultraviolet and MMS treatment. Remarkably, the 3A mutation significantly blocked the decrease of Smurf1 and the corresponding increase of RhoB induced by ultraviolet and MMS in both HeLa and HCT116 cells ( Fig. 8g,h and Supplementary Fig. 16a,b ). Accordingly, Smurf1-3A showed a more prominent effect on attenuating the apoptosis caused by ultraviolet and MMS than wild-type Smurf1 ( Fig. 8i and Supplementary Fig. 16c ). In addition, we confirmed that the Smurf1-3A has the same activity to target RhoB for degradation ( Supplementary Fig. 16d ). Taken together, our results demonstrated a novel ATR/Chk1/Smurf1 signalling pathway in determining cell fate after DNA damage by mediating RhoB abundance. ATR/Chk1 signalling pathway controls a wide range of cellular responses to DNA damage from cell cycle arrest, DNA repair, to apoptosis. The underlying mechanism for ATR/Chk1-regulated apoptosis in the DNA damage response still remains unclear [53] . In this study, we defined a novel pathway in which activation of ATR/Chk1 signalling after DNA damage promotes Smurf1 self-degradation by inducing its phosphorylation, thereby releases RhoB from the control of Smurf1 to promote apoptosis, providing another piece of the clue to elucidate the signalling network of ATR/Chk1 in regulation of apoptosis under DNA damage stress. Interestingly, cisplatin and Dox have less potency to activate Chk1 compared with ultraviolet and MMS, although they could effectively activate Chk2 ( Supplementary Fig. 12 ); therefore, treatment of cisplatin or Dox did not affect either Smurf1 or RhoB protein levels ( Supplementary Fig. 5c,d ), which is in good agreement with our finding that Smurf1 specifically interacts with Chk1 but not Chk2 and self-degradation of Smurf1 promoted by Chk1 after ultraviolet or MMS treatment is necessary for the upregulation of RhoB. Thus, our results demonstrated that Smurf1 is a downstream effector specific for ATR/Chk1 signalling in the DNA damage response. Unlike RhoA and RhoC that are relatively stable, RhoB is a short-lived protein with half-life of 2.5 h (ref. 54 ), and its levels can be quickly and transiently upregulated by various growth and stress stimuli including DNA damage [46] , [51] , [55] , [56] , [57] . However, the identity of the responsible E3 ubiquitin ligase(s) for RhoB turnover had been elusive. Our study, for the first time, identified Smurf1 as an E3 ubiquitin ligase responsible for RhoB degradation. We demonstrate here that Smurf1 plays a pivotal role in controlling RhoB abundance, which might be necessary for normal cell growth in the basal state, and ensure a prompt response to apoptosis stimuli by quickly upregulating RhoB through shutting down the Smurf1-mediated RhoB degradation. Of note, Smurf1 may have multifaceted functions in regulating apoptosis. Previous study showed that Smurf1 and Smurf2 promote p53 degradation by stabilizing MDM2, an E3 ligase for p53, therefore inhibit apoptosis [58] . Our recent study presented that under cAMP/PKA signalling, Smurf1 targets orphan nuclear receptor Nur77 for atypical ubiquitination, therefore prevents its degradation, which is required for cisplatin-induced apoptosis [49] . Together with the Smurf1-mediated RhoB degradation in the regulation of apoptosis, these studies suggest that Smurf1 may exert distinct roles in mediating apoptosis under different circumstances; however, the underlying mechanism remains to be fully understood. It is well established that defects in apoptosis may lead to tumorigenesis [59] . Interestingly, recent studies showed that Smurf1 is frequently overexpressed in various types of human cancers including colorectal and pancreatic cancers and act as a protooncoprotein [18] , [19] , [20] , [60] . Previous studies showed that Smurf1-mediated RhoA degradation is essential for TGFβ-induced epithelial-to-mesenchymal transition and cancer cell invasive activity [12] , [13] , [25] , and Smurf1 could monoubiquitinate TRAF4 to promote breast cancer cell migration [16] , indicating that Smurf1 is required for tumour malignancy. Nevertheless, the fundamental role of Smurf1 in tumorigenesis still remains largely unknown. It is noteworthy that RhoB is recognized as a tumour suppressor by virtue of its specific capability to induce apoptosis of transformed cells [46] , and loss of RhoB is found in various types of cancer [31] , [32] , [33] , [34] , [35] . Our study demonstrates a pivotal role of Smurf1 in favoring cell survival under certain DNA damage, suggesting that Smurf1 may function as an oncoprotein by excessively suppressing RhoB protein levels in tumour initiation as well. It would be of great interest to further explore the role of Smurf1-mediated RhoB degradation in tumorigenesis, which may provide us new insights into tumour development and potential strategy for cancer therapy. DNA constructs Human Smurf1 (wild-type, C699A and truncated mutants), Smurf2 (wild-type and C716A) and RhoA (wild-type and K6,7R mutant) have been previously described [12] , [13] , [47] . Human RhoB and RhoC were cloned from HEK293T cells using reverse transcription PCR. Human Chk1 and Chk2 were generous gifts from Dr S.C. Lin. RhoB-K6,7R mutant, kinase-dead Chk1-D130A mutant and non-phospho-mimicking mutant Smurf1-3A (Thr145A, Thr161A and Thr682A) were generated by PCR-based site-directed mutagenesis. Expression plasmids for various proteins were constructed into a modified pCMV5 vector for transfection or pBOBI vector for lentivirus infection. For gene silencing, the lentivirus-based vector pLL3.7 was used for expression of shRNA. The sequences used for Smurf1 shRNA-1 and -2 are 5′-GGTTACACCACATCATGAA-3′ and 5′-TGAAGGAACGGTGTATGAA-3′, respectively; for RhoB shRNA-1 and -2 are 5′-CCATCATCCTGGTGGCCAA-3′ and 5′-GCAAGACGTGCCTGCTGAT-3′, respectively; for RhoA shRNA is 5′-AAGGCAGAGATATGGCAAACA-3′; for ATM and ATR shRNA are 5′- GAAGGAAGCCAGAGTACAA-3′ and 5′-GGTCAGCTGTCTACTGTTA-3′, respectively; for Chk1 shRNA-1 and -2 are 5′-GCGTGCCGTAGACTGTCCA-3′ and 5′-AAGGGATAACCTCAAAATCTC-3′, respectively; for Chk2 shRNA-1 and -2 are 5′-GCCTTAAGACACCCGTGGC-3′ and 5′-GAGGACTGTCTTATAAAGATT-3′, respectively. The scramble sequence 5′-TTCTCCGAACGTGGCACGA-3′ was used for a control shRNA. Antibodies and chemical reagents Mouse anti-HA (sc-7392, 1:2,000), anti-Myc (sc-40, 1:2,000), anti-GFP (sc-9996, 1:2,000), anti-Ub (sc-8017, 1:1,000), anti-GST (sc-138,:2,000), anti-RhoA (sc-418, 1:2,000), anti-RhoB (sc-8048, 1:2,000), anti-GAPDH (sc-32233, 1:2,000), rabbit anti-RhoB (sc-180, 1:1,000) antibodies were purchased from Santa Cruz Biotechnology (Santa Cruz, CA, USA); mouse anti-FLAG M2 (1:2,000) antibody was purchased from Sigma; rabbit anti-Chk1 (#2345, 1:1,000), anti-Chk2 (#2662, 1:1,000), anti-Phospho-Chk1 (ser345, #2348, 1:1,000), anti-Phospho-Chk2 (Thr68, #2661, 1:1,000), anti-Phospho-Threonine (#9381, 1:1,000) antibodies were purchased from Cell Signaling Technology; rabbit anti-Phospho-serine (61-8100, 1:1,000) antibody was purchased from Invitrogen (Grand Island, NY, USA); mouse anti-Smurf1 (ab57573, 1:1,000), rabbit anti-Smurf2 (ab53316, 1:1,000) antibodies were purchased from Abcam; rabbit anti-ATM (PC116, 1:500), anti-ATR (PC538, 1:1,000) antibodies were purchased from Calbiochem; rat anti-HA monoclonal (1:2,000) antibody was purchased from Roche (Mannheim, Germany). Inhibitors for Chk1 (UCN-01, #539644) and Chk2 (Chk2 inhibitor-II #220486) were purchased from Calbiochem; proteasome inhibitor MG-132 was from Boston Biochem (Cambridge, MA, USA); chloroquine, MMS, Dox, cisplatin, actinomycin D, cycloheximide and Caffeine were from Sigma (St Louis, MO, USA). Cell culture and transfection Human embryonic kidney HEK293T, human cervical cancer HeLa, mink lung epithelial Mv1Lu, human breast cancer MCF-7, human lung adenocarcinoma A549, human hepatocellular carcinoma HepG2, mouse fibroblast NIH3T3 and mouse embryonic fibroblast cells were cultured in high-glucose Dulbecco’s modified Eagle’s medium, human colorectal carcinoma HCT116, human colon cancer SW480, human colon cancer HT-29 and human osteosarcoma U2OS cells were cultured in McCoy’s 5A medium, all supplemented with 10% (v/v) fetal calf serum (Gibco) and 100 units ml −1 streptomycin and penicillin (Millipore, Billerica, MA, USA), at 37 °C in a humidified 5% CO 2 incubator. HEK293T, HeLa, A549, U2OS, HepG2, Mv1Lu, SW480 and NIH3T3 cells were obtained from ATCC. HCT116, HT-29 and MCF-7 cells were purchased from the Cell Bank of the Chinese Academy of Sciences (Shanghai). Mouse embryonic fibroblast cells were a kind gift from Dr J Han. HEK293T cells were transiently transfected using a calcium–phosphate method as previously described [61] . Mv1Lu cells were transiently transfected with Lipofectamine 2000 (Invitrogen) following the manufacturer’s protocol. Recombinant lentivirus was generated using the ViraPower Lentiviral Expression System (Invitrogen) for infecting HeLa and HCT116 cells. IP and IB assays IP and IB assays were performed as previously described [61] . Briefly, cells were lysed on ice with lysis buffer TNTE 0.5% (50 mM Tris–HCl, pH 7.5, 150 mM NaCl, 1 mM EDTA and 0.5% Triton X-100, containing 10 μg ml −1 pepstatin A, 10 μg ml −1 leupeptin and 1 mM PMSF). The cell lysates were applied to IP or IB assays with appropriate antibodies. All the uncropped scans of the most important immunoblots are included in Supplementary Figs 17–21 . Ubiquitination and GST pull-down assays Ubiquitination and GST pull-down assays were also performed as previously described [61] . For in vivo ubiquitination assay, cell lysates were subjected to anti-Flag IP, eluted by boiling 5 min in 1% SDS, diluted 10 times in lysis buffer TNTE 0.5% and then re-immunoprecipitated with anti-Flag (2 × IP). The ubiquitin-conjugated proteins were detected by IB. For GST pull-down and in vitro ubiquitination assays, bacterially expressed GST/Smurf1 (WT, C699A or truncated mutants) and GST/RhoB were purified using glutathione sepharose beads in TNTE 0.5% buffer. Free RhoB proteins were obtained by TEV protease cleavage. Immunofluorescence assay Twenty-four hours after transfection, cells grown on glass coverslips were washed three times in phosphate-buffered saline (PBS), fixed with 4% paraformaldehyde and permeabilized with 0.25% Triton X-100, then stained using appropriate primary and fluorescently conjugated secondary antibodies. Flag-tagged Rho proteins were detected using mouse anti-Flag M2 antibody followed by Alexa Fluor 555 or 647-conjugated donkey anti-mouse secondary antibody (Invitrogen), and HA-tagged Smurf1 was stained using rat anti-HA antibody followed by Alexa Fluor 488-conjugated donkey anti-rat secondary antibody (Invitrogen). Texas Red conjugated Phalloidin was used for F-actin staining. Images were obtained using a ZEISS LSM 780 confocal microscope with ZEN 2010 software (Carl Zeiss GmbH, Jena, Germany). Ultraviolet irradiation and MMS treatment Cells at 50–70% confluence were exposed to 80 J m −2 or 10 J m −2 of ultraviolet in Spectrolinker XL-1000 (Spectronics) without culture medium, followed by incubation in the original medium for determined time. For MMS treatment, cells were treated with 0.5 mM MMS for determined time and then subjected to IB or flow cytometry. Apoptosis assay Cells cultured in 12-well plates were treated with ultraviolet or MMS, trypsinized and collected. The cells were washed in PBS and fixed with 70% ethanol overnight, washed and incubated in PBS with 100 units ml −1 RNaseA at 37 °C for 30 min, and then stained with 50 μg ml −1 propidium iodide in PBS for 30 min at 37 °C in the dark. The percentages of apoptotic cells were calculated by determining sub-G1 proportion of cells using a Beckman Coulter Epics XL flow cytometer (Beckman Coulter, Indianapolis, IN, USA). In vitro kinase assay HEK293T cells transfected with triple Flag-tagged wild-type Chk1 or its dominant-negative form Chk1-D130A were pretreated with MMS (0.5 mM) for 2 h to active the Chk1 before subjected to IP with Flag antibody and Protein G agarose beads, followed by washing twice with 0.5% TNTE and twice with kinase reaction buffer (20 mM Tris–HCl pH 7.5, 10 mM MgCl 2 , 1 mM dithiothreitol, 25 μM ATP). GST/Smurf1 or its mutants purified from bacteria were incubated with Chk1-bound agarose beads in a total volume of 20 μl of reaction buffer at 30 °C for 30 min before subjected to IB assay. Subcellular fractionation Cells were washed twice with ice-cold PBS before lysed in ice-cold buffer A (10 mM HEPES pH 7.9, 1.5 mM MgCl 2 , 10 mM KCl, 1 mM DTT, 0.5 mM PMSF, 0.1% NP-40) for 10 min and then centrifuged at 1,200 r.p.m. for 5 min. The clear cytoplasmic fraction was collected by recentrifuging the supernatant at 12,000 r.p.m. for 10 min. The nuclear fraction was obtained by washing the nuclei-containing pellet with cold PBS and resuspended in buffer B (10 mM HEPES pH 7.9, 20% glycerol, 0.3 M NaCl, 1.5 mM MgCl 2 , 0.4 mM EDTA, 0.5% NP-40, 1 mM DTT, 0.5 mM PMSF) on a rotator at 4 °C for 30 min and then centrifuged at 12,000 r.p.m. for 10 min. Quantitative RT–PCR Total RNAs were extracted from cells or tissue samples using Trizol reagent (Invitrogen) according to the manufacturer’s instructions. Reverse transcription was performed with 500 ng of total RNA using PrimeScript High Fidelity Reverse Transcriptase kit (Takara, Dalian, China). Real-time amplification of transcripts was performed using a Mastercycler EP gradient S RealPlex2 (Eppendorf, Hamburg, Germany). The relative changes of gene expression were determined using the 2 −ΔΔCt method by normalizing to the internal control gene GAPDH. The primers for RhoB are 5′-GCAGCGACGAGCATGTCC-3′ (forward) and 5′-CCGTTCTGGGAGCCGTAG-3′ (reverse); for Smurf1 are 5′-AGATCCGTCTGACAGTGTTATG-3′ (forward) and 5′-CCCATCCACGACAATCTTTGC-3′ (reverse); and for GAPDH are 5′-CATGAGAAGTATGACAACAGCCT-3′ (forward) and 5′-AGTCCTTCCACGATACCAAAGT-3′ (reverse). Statistical analysis One-way analysis of variance with Tukey’s HSD post test was used to compare values between different experimental groups using the SPSS Statistics 19.0 programme. P <0.05 was considered a statistically significant change, * P <0.05, ** P <0.01 and *** P <0.001. All the values were presented as means±s.d. of at least triplicate experiments. How to cite this article : Wang, M. et al. ATR/Chk1/Smurf1 pathway determines cell fate after DNA damage by controlling RhoB abundance. Nat. Commun. 5:4901 doi: 10.1038/ncomms5901 (2014).